Restricted perinatal retinal degeneration induces retina reshaping and correlated structural rearrangement of the retinotopic map The formation of the retinotopic map depends on the action of axon guidance molecules, activity-dependent mechanisms and axonal competition. However, little is known about the plasticity potential of the system and the effects on the remodelling of retinocollicular connections upon retinal insults. Here we create a mouse model in which retinal ganglion cells that project to anterior and posterior superior colliculus undergo cell death during topographic map formation. We show that the remaining retinal ganglion cells expand the targeted area in the superior colliculus and at the same time increase their spatial coverage in the retina in a correlated fashion. The resulting contralateral topographic map is overall maintained but less precise, while ipsilateral retinal ganglion cell axons are abnormally distributed in anterior and posterior superficial superior colliculus. These results suggest the presence of plastic mechanisms in the developing mammalian visual system to adjust retinal space and its target coverage and ensure a uniform map. A fundamental principle in the generation of sensory connectivity is its arrangement in topographic maps. The visual system has largely served as a model to identify the molecules and mechanisms critical for the formation of such maps [1] . In mouse, retinal ganglion cell (RGC) axons initially overshoot their target in the superior colliculus (SC) and subsequently refine their terminations to the topographically appropriate locations, mapping the temporal–nasal and the dorsal–ventral retinal axes along the anterior–posterior and lateral–medial collicular axes, respectively [2] . The remodelling of the initial axon overshoot during the first postnatal week depends on the combined actions of axon guidance molecules, activity-dependent mechanisms and axon competition [1] , [3] , [4] . About 95% of the RGCs project to the contralateral SC and terminate in the dorsal-most layer (stratum griseum superficiale, SGS), whereas 5% of RGCs axons, originating in the temporal–ventral crescent (VTC) of the retina, stay ipsilaterally and target the stratum opticum (SO), a deeper layer of the SC [5] , [6] . Historically, two main technical approaches have been considered to study the role of competition for correct retinotopic map formation: retinal ablation/enucleating studies or mutant models with uniformly decreased numbers of RGCs. Studies in amphibia and fish described that RGC axons can fill available space in the optic tectum after retinal lesions [7] , [8] , [9] . However, in contrast to mammals, these species exhibit retinal regenerative properties, making direct comparisons difficult [10] . Pioneering studies in neonatal rodents using retinal enucleation or raw mechanical lesions revealed that remaining RGC axons are able to expand into depleted areas of the SC [11] , [12] . Interestingly, different studies suggest that axon competition is important for topographic map formation in mouse [13] , but not in zebrafish [14] . However, it is not clear to date if a localized retinal insult in mammals leads to an organizational change of the remaining cells in the eye, and if so, what are the consequences for topographic map formation. For this purpose, we created a genetic degeneration mouse model in which the nasal and temporal retina undergoes cell death during the perinatal period. We used a mouse line containing a floxed allele of Dicer1 (Dicer fl/fl ) [15] in combination with a line expressing the Cre-recombinase under the control of the Pax6-α promoter element (αCre) [16] . Crosses between these lines lead to the specific deletion of Dicer in retinal progenitor cells in nasal and temporal retina [17] , [18] . The deletion of Dicer1 in neuronal progenitors, but not in differentiated neurons, leads to cell death [19] , [20] , [21] , [22] . As a consequence, we eliminate projections from nasal and temporal retina without affecting any other areas. We present here the creation of a mammalian model system with a reproducible genetic retinal lesion to study retinal plasticity and RGC axon competition during topographic map development. Upon lesion, we find a rearrangement of the remaining RGCs in the retina and, at the same time, targeting changes of their axons along ipsi- and contralateral pathways. Our results suggest the presence of correlated plastic mechanisms to adjust retinal space and its coverage in the target to ensure a uniform retinotopic map. Partial retinal degeneration affects remaining RGC projections To investigate the effect of an early genetic retinal lesion on the formation of retinocollicular connectivity, we generated a genetic mouse model in which a defined part of the retina degenerates during the time window of retinotopic map formation [2] . We used mice carrying a conditional allele (floxed, fl) of the ribonuclease Dicer1 (ref. 15 ) in combination with a line expressing the Cre-recombinase under the control of the Pax6α−promoter element (αCre) [16] . This leads to the specific deletion of Dicer1 in retinal progenitor cells in distal areas of nasal and temporal retina, starting at embryonic day (E)10.5. As a consequence, these areas show severe defects in retinal morphogenesis and, at postnatal stages, result in thin retinal areas consisting mainly of retinal and ciliary body progenitors, with only few misplaced RGCs without axons at postnatal day (P)8 ( Fig. 1 ) [17] , [18] . In contrast, the Cre-negative retinal area remains unaffected ( Fig. 1b ). To identify Cre-positive cells, we generated crosses in the background of a reporter line, expessing EYFP upon Cre-mediated deletion of a stop-cassette (R26R-EYFP) [23] . Retinal sections of mutant (αCre;Dicer fl/fl ;R26R-EYFP) and heterozygous control (αCre;Dicer fl/+ ;R26R-EYFP) mice show, at P0, EYFP-positive RGCs located in distal nasal and temporal retina with their axons exiting the retina through the optic disc, projecting towards the chiasm and finally innervating the SC ( Fig. 1a and Supplementary Fig. S1 ). At P8, however, when retinotopic map refinement is complete, no EYFP-positive axons can be detected anymore in mutant mice at the optic disc ( Fig. 1c ) or in the SC (not shown). To visualize the remaining wild-type axons, we filled each eye with distinguishable anterograde axon tracers, choleratoxin B-subunit (CTB), conjugated to red (Alexa-594) or green (Alexa-488) fluorophores. We found that in mutants the optic nerve, although present, is dramatically reduced in size at P8 compared with wild-type littermates ( Fig. 1e ). Immunohistochemical detection showed a significant increase of Caspase-3-positive cells in nasal and temporal Cre-positive retinal areas in mutant mice, confirming retinal degeneration during the time of visual map maturation ( Supplementary Fig. S2 ) [18] . The Cre-recombinase is also expressed in a subset of committed or already differentiated amacrine cells across the retina, which does not affect their survival [24] . 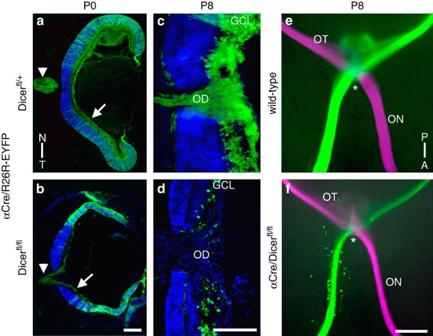Figure 1: Retinal Dicer1-deletion leads to lamination defects and RGC degeneration. Cryosections of heterozygous control (a,c) and mutant (b,d) eyes and subsequent immunohistochemical analysis using anti-GFP (green) antibodies to visualize Cre-positive cells and DAPI counterstain (blue). (a,b) Retinal lamination and thickness are already affected at P0 in Dicer-deleted nasal and temporal retinal areas (b), but EYFP-positive axons coming from nasal and temporal peripheral retina are still present in the fibre layer (arrow) and in the optic nerve (arrowheads). (c,d) Higher magnifications of the optic discs (OD) in control (c) and mutant (d) mice at P8. In contrast to the controls (c), Dicer-negative (EYFP+) RGC axons have disappeared in mutant mice and no longer exit the OD (d). (e,f) Ventral whole-mount view of the optic chiasm (asterisks) under fluorescent illumination after full eye injections of CTB-Alexa-594 and 488 at P8. Wild-type mice show normal sized optic nerves (ON) and optic tracts (OT) (e). In contrast, mice with degenerated nasal and temporal retinal areas exhibit thinner ON and OT, but still forming a normal chiasm at the ventral midline (f). A–P; anterior–posterior; GCL, ganglion cell layer; N–T, nasal–temporal. Scale bar, 200 μm. Figure 1: Retinal Dicer1-deletion leads to lamination defects and RGC degeneration. Cryosections of heterozygous control ( a , c ) and mutant ( b , d ) eyes and subsequent immunohistochemical analysis using anti-GFP (green) antibodies to visualize Cre-positive cells and DAPI counterstain (blue). ( a , b ) Retinal lamination and thickness are already affected at P0 in Dicer-deleted nasal and temporal retinal areas ( b ), but EYFP-positive axons coming from nasal and temporal peripheral retina are still present in the fibre layer (arrow) and in the optic nerve (arrowheads). ( c , d ) Higher magnifications of the optic discs (OD) in control ( c ) and mutant ( d ) mice at P8. In contrast to the controls ( c ), Dicer-negative (EYFP+) RGC axons have disappeared in mutant mice and no longer exit the OD ( d ). ( e , f ) Ventral whole-mount view of the optic chiasm (asterisks) under fluorescent illumination after full eye injections of CTB-Alexa-594 and 488 at P8. Wild-type mice show normal sized optic nerves (ON) and optic tracts (OT) ( e ). In contrast, mice with degenerated nasal and temporal retinal areas exhibit thinner ON and OT, but still forming a normal chiasm at the ventral midline ( f ). A–P; anterior–posterior; GCL, ganglion cell layer; N–T, nasal–temporal. Scale bar, 200 μm. Full size image The degeneration in nasal and temporal retina results in a remaining central region of Cre-negative RGCs along the dorsal–ventral axis. This area projects and terminates, according to the normal topographic map, to a region in the central SC along its medial–lateral axis [2] . This area can be visualized in mice containing both the αCre and R26R-EYFP alleles (EYFP-negative area in Fig. 2a ). We next tested if the removal of axon terminations in anterior and posterior SC (caused by the genetically induced temporal and nasal retinal lesion, respectively) influences the targeting of the remaining axons. To analyse the area innervated by the wild-type RGCs, we filled each eye of α-Del mutant mice with CTB-Alexa-594 or -488. We hypothesized that without plasticity potential during visual map remodelling and upon loss of nasal and temporal RGCs, the remaining wild-type RGC axons should terminate only at their topographically appropriate central position in the SC ( Fig. 2b , left). In contrast, if the system allows for plasticity, the terminations should expand anterior- and posteriorly ( Fig. 2b , right). Consistent with the latter option, we found a substantial expansion of terminations from wild-type RGCs in the contralateral SC of α-Del mice at P8, although the extreme anterior and posterior zones remained empty ( Fig. 2c ). Interestingly, we detected in all cases small patches generated by axons from the ipsilateral eye in anterior and posterior locations, completely segregated from the contralateral terminations ( Fig. 2c inset). This aberrant phenotype was already detectable during map refinement at P4, and remained stable, as analysis of the retinopic map at P14 and after eye opening at P21 did not show any change ( Supplementary Fig. S3 ). In control mice, anterograde labelling from both eyes filled the entire SCs, containing no superficial ipsilateral patches ( Fig. 2c ). These findings validate the α-Del mutant mouse as a tool to study plasticity of neural projections in the visual system upon the loss of cells in defined retinal domains at perinatal ages. 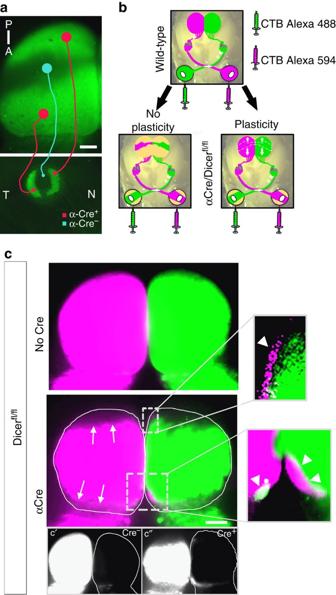Figure 2: Retinal degeneration results in an extension of the remaining retinocollicular projections. (a) Dorsal view of the SC (upper panel) and retina (lower panel) at P8 of a αCre+;Dicer+/fl;R26R-EYFP mouse illustrating the Cre-positive areas (green) in the retina and their termination areas in the SC. Nasal (N) and temporal (T) retinal areas map onto posterior (P) and anterior (A) SC, respectively (red lines), whereas the central retina (Cre-negative) maps onto the central SC (blue line). (b) Schematic describing possible outcomes of mapping behaviour of axons originating in remaining central retina, after degeneration of nasal and temporal areas. Without any plasticity (left panel), the RGC axons should map according to their topographic labels and the labelled SC area should thus be confined to the central area, similar to the Cre-negative area shown in (a). If plasticity is involved (right panel) an extension of the labelled area towards anterior and posterior SC is expected. (c) Dorsal view of the SC at P8 of a wild-type (upper panel) and α-Del mouse (lower panel) after full eye fills with CTB-Alexa-488 (green) and -594 (magenta). In wild-type mice, both colliculi are filled completely with axon terminations from the contralaleral eye. In contrast, mice with nasal and temporal degenerations exhibit an incomplete fill of the SC by the projections from contralateral RGCs, leaving some areas at the anterior and posterior end empty (arrows). In addition, small zones occupied by RGC axons originating from the ipsilateral retina are visible in each anterior and posterior SC (arrowheads, boxed areas and higher magnifications). Single channel images (Alexa-594) are shown in c′ and c′′ for increased contrast and signal detection. A–P, anterior–posterior; N–T nasal–temporal. Scale bar, 200 μm. Figure 2: Retinal degeneration results in an extension of the remaining retinocollicular projections. ( a ) Dorsal view of the SC (upper panel) and retina (lower panel) at P8 of a αCre + ;Dicer +/fl ;R26R-EYFP mouse illustrating the Cre-positive areas (green) in the retina and their termination areas in the SC. Nasal (N) and temporal (T) retinal areas map onto posterior (P) and anterior (A) SC, respectively (red lines), whereas the central retina (Cre-negative) maps onto the central SC (blue line). ( b ) Schematic describing possible outcomes of mapping behaviour of axons originating in remaining central retina, after degeneration of nasal and temporal areas. Without any plasticity (left panel), the RGC axons should map according to their topographic labels and the labelled SC area should thus be confined to the central area, similar to the Cre-negative area shown in ( a ). If plasticity is involved (right panel) an extension of the labelled area towards anterior and posterior SC is expected. ( c ) Dorsal view of the SC at P8 of a wild-type (upper panel) and α-Del mouse (lower panel) after full eye fills with CTB-Alexa-488 (green) and -594 (magenta). In wild-type mice, both colliculi are filled completely with axon terminations from the contralaleral eye. In contrast, mice with nasal and temporal degenerations exhibit an incomplete fill of the SC by the projections from contralateral RGCs, leaving some areas at the anterior and posterior end empty (arrows). In addition, small zones occupied by RGC axons originating from the ipsilateral retina are visible in each anterior and posterior SC (arrowheads, boxed areas and higher magnifications). Single channel images (Alexa-594) are shown in c′ and c′′ for increased contrast and signal detection. A–P, anterior–posterior; N–T nasal–temporal. Scale bar, 200 μm. Full size image Remodelling of the retina after induced partial degeneration To investigate whether the expanded RGC axon terminations in the SC are accompanied by a morphological rearrangement of the remaining retina, we analysed the eyes of mice affected by the degeneration before and after retinocollicular map formation. We found that upon Dicer1-deletion, small morphological changes in peripheral retinal domains are already evident on sections at birth ( Fig. 1 ) [17] , [18] . At P8, the mutant retinae display further thinning at distal positions, described in previous reports as ciliary margin-like areas [17] . We noticed, however, that the relative extent of these degenerated distal areas was much smaller than expected, suggesting an expansion of the Cre-negative central retinal domain in mutant mice (curved lines in Fig. 3a ). We therefore measured the area of the Cre-negative (EYFP-negative, wild-type) retinal tissue in relation to the total retinal size and calculated a relative Cre-negative index at P8 ( Fig. 3g ). Although the absolute size of mutant retinae was smaller than in wild-type littermates (8.6±0.2 mm 2 versus 12.1±0.3 mm 2 , respectively, n =8 for each genotype), the proportion of retinal area occupied by Cre-negative cells was significantly larger in mutants (7.3±0.1 mm 2 or 0.85±0.02), compared with wild-type (2.7±0.1 mm 2 or 0.22±0.02). Interestingly, this corresponds perfectly with the expansion of the targeted area in the SC by Cre-negative RGCs in mutant mice versus wild-type mice (0.84±0.04, n =9; 0.23±0.01, n =8, respectively, Fig. 3i ). These changes were already evident from the onset of the retinal degeneration at P0 ( Supplementary Fig. S4 ). 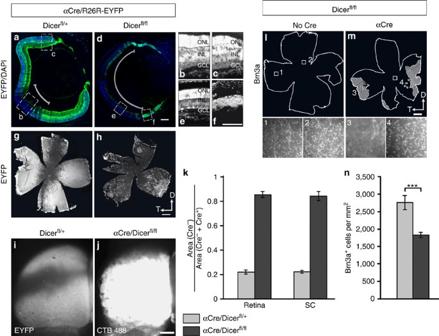Figure 3: Genetic retinal lesions induce an expansion of the central retina and RGC projections in the SC. (a–h) Immunohistochemical detection of EYFP+ (Cre+, green) regions on cryosections (a,d) and flat mounts (g,h) in heterozygous controls and homozygous mutant retinae at P8, counterstained with DAPI (blue). Mutant retinae have an enlarged Cre-negative domain compared with wild-type or heterozygous control animals (curved lines in a,d). (b,c,e,f) Retinal lamination is the same for regions outside (b) and inside (c) the Cre-positive areas in control animals, but differs significantly in mutant mice presenting a normal lamination outside (e), but only a single thin layer of cells in the distal Cre-positive areas (f). (i) Dorsal view of a SC at P8 of control animals, stained against EYFP. The central EYFP-negative domain illustrates the area free of temporal and nasal RGC projections. (j) Dorsal view of a SC at P8 after full fills of the contralateral eye with CTB Alexa-488. RGC axons avoid the most anterior and posterior SC domains. (k) Relative Cre-negative index in retina and SC of control and α-Del mutant mice. Quantification shows that in control mice the Cre-negative index is 0.2 in both retina and SC (n=8 retinae and SCs, same animals). In contrast, in mutant mice this index reaches values above 0.8%, but stays correlated between retina and SC (n=8 retinae,n=9 SCs, different animals). (l,m) Immunohistochemical detection of Brn3a-positive cells in retinae from α-Del mutant and Cre-negative control mice at P8. Insets (1–4) illustrate Brn3a-positive cells in central and peripheral retina as shown in the camera lucida schematics. (n) Density quantification of Brn3a-positive cells for both genotypes. Unpaired Student’st-test. (k,n) Values are mean±s.e.m. D, dorsal; GCL, ganglion cell layer; INL, inner nuclear layer; ONL, outer nuclear layer; T, temporal. Scale bar, 500 μm (g,h,l,m) and Scale bar, 200 μm (a,d,i,j). Figure 3: Genetic retinal lesions induce an expansion of the central retina and RGC projections in the SC. ( a – h ) Immunohistochemical detection of EYFP+ (Cre+, green) regions on cryosections ( a , d ) and flat mounts ( g , h ) in heterozygous controls and homozygous mutant retinae at P8, counterstained with DAPI (blue). Mutant retinae have an enlarged Cre-negative domain compared with wild-type or heterozygous control animals (curved lines in a,d). ( b , c , e , f ) Retinal lamination is the same for regions outside ( b ) and inside ( c ) the Cre-positive areas in control animals, but differs significantly in mutant mice presenting a normal lamination outside ( e ), but only a single thin layer of cells in the distal Cre-positive areas ( f ). ( i ) Dorsal view of a SC at P8 of control animals, stained against EYFP. The central EYFP-negative domain illustrates the area free of temporal and nasal RGC projections. ( j ) Dorsal view of a SC at P8 after full fills of the contralateral eye with CTB Alexa-488. RGC axons avoid the most anterior and posterior SC domains. ( k ) Relative Cre-negative index in retina and SC of control and α-Del mutant mice. Quantification shows that in control mice the Cre-negative index is 0.2 in both retina and SC ( n =8 retinae and SCs, same animals). In contrast, in mutant mice this index reaches values above 0.8%, but stays correlated between retina and SC ( n =8 retinae, n =9 SCs, different animals). ( l , m ) Immunohistochemical detection of Brn3a-positive cells in retinae from α-Del mutant and Cre-negative control mice at P8. Insets ( 1 – 4 ) illustrate Brn3a-positive cells in central and peripheral retina as shown in the camera lucida schematics. ( n ) Density quantification of Brn3a-positive cells for both genotypes. Unpaired Student’s t -test. ( k , n ) Values are mean±s.e.m. D, dorsal; GCL, ganglion cell layer; INL, inner nuclear layer; ONL, outer nuclear layer; T, temporal. Scale bar, 500 μm ( g , h , l , m ) and Scale bar, 200 μm ( a , d , i , j ). Full size image We next determined the number of RGCs to calculate their density in the mutant retinae. As the Cre-negative RGCs expanded their retinal coverage in mutant mice, we expected a lower density than in wild-type mice. For this, we used detection of Brn3a, a common marker labelling about 80% of all RGCs [25] , on whole-mount retinae ( Fig. 3 l ). At P0, RGCs were still present in Cre-positive domains of mutant animals ( Supplementary Fig. S4 ), as seen before ( Supplementary Fig. S1 ). At this early stage the total number of RGCs (Brn3 + cells) in the Cre-negative zone of lesioned mutant retinae is similar to wild-type (30,166±2,984 versus 29,679±4,160, n =4 for each genotype). The small area increase seen at P0 ( Supplementary Fig. S4 ) therefore leads to a slight decrease in cell density in the Cre-negative domain of the mutant retina compared with wild-type (12,569±695 RGCs per mm 2 versus 15,547±463 RGCs per mm 2 , respectively). At P8, when all Cre-positive RGCs initially sending out axons have degenerated, we find that in mutant mice the density of the remaining RGCs is now strongly reduced (1,909 ±96 RGCs per mm 2 , n =5) compared with wild-type littermates (2,876±239 RGCs per mm 2 , n =5) ( Fig. 3n ). Interestingly, although the total number of RGCs in the lesioned mutant retinae was smaller compared with controls (13,995±839 versus. 34,800±2,127 RGCs, n =5 for both genotypes), we detected significantly more Cre-negative Brn3+ cells in mutants than in wild-type mice (13,995±839 versus 7,656±1,258 RGCs, respectively). As in mice normally more than half of all RGCs die between P2 and P5 (ref. 26 ), this detected increase could have two possible reasons: a decrease in cell death and/or an increase in cell proliferation. To distinguish between these possibilities, we used specific markers for both processes. Immunohistochemical detection of Caspase-3 showed indeed a 50% drop of apoptotic cells in the RGC layer within the Cre-negative areas of lesioned mutant retinae at P3 ( Fig. 4a–c ). In contrast, detection of Ki67, a marker for cell proliferation, showed no differences in these areas between genotypes ( Fig. 4d–h ). 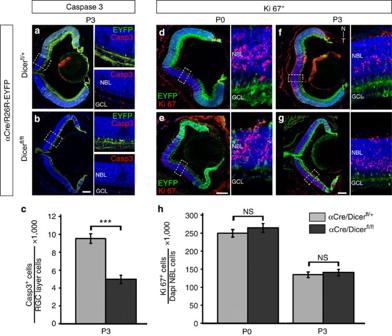Figure 4: Postnatal mutant lesioned retinae involves alterations in cell death rate. Immunohistochemical detection of EYFP (green) and Caspase-3 (red) on P3 retina cryosections from control heterozygous (a) and α-Del mutant (b) mice, counterstained with the nuclear marker DAPI (blue). High magnification of boxed areas in (a,b) are shown to the right. (c) Quantification shows a 50% reduction of apoptotic cells in Cre-negative parts of the RGC layer of mutant mice, compared with control littermates. (d–h) Immunohistochemical detection of EYFP (green) and proliferation marker Ki67 (red) on retina cryosections from control heterozygous (d,f) and mutant (e,g) mice, counterstained with the nuclear marker DAPI (blue). Both, at P0 (d,e) and P3 (f,g), the number of proliferating cells in the neuroblastic layer (NBL) of Cre-negative retinal areas is similar between mutant and control littermates. High magnifications of boxed areas are shown to the right. Quantifications are shown in (h). Values in (c,h) are mean±s.e.m; five fields for each different embryo (four embryos for each test) were analysed. Unpaired Student’st-test ***P<0.001, NS, not significant;P>0.2. GCL, ganglion cell layer; N–T, nasal–temporal. Scale bar, 200 μm. Figure 4: Postnatal mutant lesioned retinae involves alterations in cell death rate. Immunohistochemical detection of EYFP (green) and Caspase-3 (red) on P3 retina cryosections from control heterozygous ( a ) and α-Del mutant ( b ) mice, counterstained with the nuclear marker DAPI (blue). High magnification of boxed areas in ( a , b ) are shown to the right. ( c ) Quantification shows a 50% reduction of apoptotic cells in Cre-negative parts of the RGC layer of mutant mice, compared with control littermates. ( d – h ) Immunohistochemical detection of EYFP (green) and proliferation marker Ki67 (red) on retina cryosections from control heterozygous ( d , f ) and mutant ( e , g ) mice, counterstained with the nuclear marker DAPI (blue). Both, at P0 ( d , e ) and P3 ( f , g ), the number of proliferating cells in the neuroblastic layer (NBL) of Cre-negative retinal areas is similar between mutant and control littermates. High magnifications of boxed areas are shown to the right. Quantifications are shown in ( h ). Values in ( c , h ) are mean±s.e.m; five fields for each different embryo (four embryos for each test) were analysed. Unpaired Student’s t -test *** P <0.001, NS, not significant; P >0.2. GCL, ganglion cell layer; N–T, nasal–temporal. Scale bar, 200 μm. Full size image In summary, we found that upon perinatal retinal degeneration, the remaining wild-type RGCs expand to cover a larger retinal area, resulting in a reduced cell density. This is counterbalanced to a certain degree with a reduction of retinal apoptosis in this area. The relative retinal area occupied upon expansion by Cre-negative RGCs matches the relative proportion of extended SC area innervated by retinal axon terminals, suggesting mechanisms to adjust retinal space and its coverage in the target in a correlated fashion. The retinotopic map is maintained but less refined Our RGC counts in the mutant retina show that only about 40% of RGCs are persisting, however, they occupy about 85% of the target. Studies in zebrafish have shown that the lack of axon competition leads to an increase of branching, but does not alter overall retinotopography [14] , whereas mice with less RGCs across the retina exhibit severe mapping defects [13] . We therefore wanted to know if in our mouse model the retinotopic map of the remaining RGCs is accurate and if branching areas of individual termination zones (TZs) are increased. For this purpose, we injected fluorescent latex beads into the SC to retrogradely label RGCs and determine their position in the retina. In wild-type mice, injections into anterior, central and posterior SC label RGCs in small foci in contralateral temporal, central and nasal retina, respectively, consistent with a normal topographic map ( Fig. 5a–c ). Our analysis of the α-Del mutant mice showed that this general pattern was conserved, when measured by the centre of mass of labelled RGCs. We noticed however, that the labelled RGCs appeared to be more spread across the retina without forming tight foci ( Fig. 5d–f ). To quantify this, we divided the retina in six concentric bins around the centre of mass and calculated the ratio between the RGCs in each peripheral circle (1–5) and RGCs found in the central circle ( Fig. 5g ). Unlike in the wild-type controls where 89.95±2.58% ( n =13) of labelled RGCs were concentrated in the centre circle, we found that in α-Del retinae the centre circle contained only 70.33±3.80% ( n =13) of labelled RGCs. In addition, we found that the ratios were significantly higher in the mutant mice than in the wild-type controls for each of the concentric bins ( Fig. 5g ). This increased spread of labelled cells was independent of retinal location and therefore applied to the entire extend of the visual map. As a complementary approach, we labelled RGC axons anterogradely and analysed their projections to the SC using the lipophilic dye DiI. Small focal injections into ventral retina result in small TZs in medial SC of P8 wild-type mice ( Fig. 5h ). In contrast, similar injections into the retinae of α-Del mutants resulted in consistently larger TZs, with many unrefined branches (arrowheads, Fig. 5i ). We also observed axons projecting and terminating outside the topographically appropriate position containing several proximal long branches, suggesting immature map refinement (arrows, Fig. 5i ). 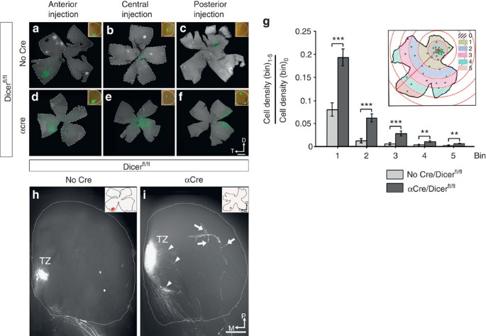Figure 5: Retinotopic map of lesion-induced expanded projections is less precise. (a–f) Whole retina flatmounts detecting RGCs after retrograde labelling using fluorescent microbeads injected in the contralateral SC of control (a–c) or lesion-induced mutant mice (d–f) at P8. Injections were made in the anterior (a,d) (n=3 for both genotypes), central (b,e) (n=4 α-Del,n=5 wild-type) and posterior (c,f) (n=6 α-Del,n=5 wild-type) SCs of mice (insets) which result in labelled RGCs in temporal, central and nasal retina, respectively. α-Del mutant mice show general conservation of the topographic map, however, exhibit larger spread of retrogradely labelled cells. (g) Quantification of spread by binning the labelled RGCs in six concentric circles (0–5), centred around the point with highest RGCs density (0). The ratio of labelled cells was calculated for each bin (1–5) in relation to the number found in the central circle (0, schematic). Retinae from α-Del mutant mice showed a significantly higher spread for each bin compared with wild-type littermates. Sample passed Kolmogov–Smirnov test. Analysis of variance followed by Bonferronipost-hoctest was applied. (n=13 for both genotypes). Values are mean±s.e.m. ***P<0.001, **P<0.01. (h,i) Dorsal view of the SC of wild-type and α-Del mice at P8 after focal DiI injections into the contralateral eye. Ventral DiI injections lead to a TZ in medial SC in both genotypes. However, the lesion-induced mutant mice show consistently larger TZs with areas of loosely organized arborizations surrounding the TZ (arrowheads). In addition, several aberrant branches outside the appropriate TZ location are detected (arrows). Insets show the position of DiI injection in the retina (n=5 wild-type,n=2 α-Del). D, dorsal; M, medial; P, posterior; T, Temporal. Scale bar, 500 μm (a–f) and Scale bar, 200 μm (h,i). Figure 5: Retinotopic map of lesion-induced expanded projections is less precise. ( a – f ) Whole retina flatmounts detecting RGCs after retrograde labelling using fluorescent microbeads injected in the contralateral SC of control ( a – c ) or lesion-induced mutant mice ( d – f ) at P8. Injections were made in the anterior ( a , d ) ( n =3 for both genotypes), central ( b , e ) ( n =4 α-Del, n =5 wild-type) and posterior ( c , f ) ( n =6 α-Del, n =5 wild-type) SCs of mice (insets) which result in labelled RGCs in temporal, central and nasal retina, respectively. α-Del mutant mice show general conservation of the topographic map, however, exhibit larger spread of retrogradely labelled cells. ( g ) Quantification of spread by binning the labelled RGCs in six concentric circles (0–5), centred around the point with highest RGCs density (0). The ratio of labelled cells was calculated for each bin (1–5) in relation to the number found in the central circle (0, schematic). Retinae from α-Del mutant mice showed a significantly higher spread for each bin compared with wild-type littermates. Sample passed Kolmogov–Smirnov test. Analysis of variance followed by Bonferroni post-hoc test was applied. ( n =13 for both genotypes). Values are mean±s.e.m. *** P <0.001, ** P <0.01. ( h , i ) Dorsal view of the SC of wild-type and α-Del mice at P8 after focal DiI injections into the contralateral eye. Ventral DiI injections lead to a TZ in medial SC in both genotypes. However, the lesion-induced mutant mice show consistently larger TZs with areas of loosely organized arborizations surrounding the TZ (arrowheads). In addition, several aberrant branches outside the appropriate TZ location are detected (arrows). Insets show the position of DiI injection in the retina ( n =5 wild-type, n =2 α-Del). D, dorsal; M, medial; P, posterior; T, Temporal. Scale bar, 500 μm ( a – f ) and Scale bar, 200 μm ( h , i ). Full size image As the accurate formation of topographic maps is dependent on the correct patterning of the retina and proper expression of guidance cues [27] , we performed in situ hybridization studies using specific riboprobes against FoxG1 , EphrinA5 and FoxD1 , EphA5, EphA6, as specific markers of nasal and temporal retina, respectively. We detected no change for any of these markers, confirming normal patterning and presence of guidance cues in our mutant retinae ( Supplementary Fig. S5 ). Together, our data using antero- and retrograde labelling suggest that the overall topographic map, although generally correct, is more diffuse in the mutant mice. This is consistent with a mechanism in which fewer cells are mapping onto a proportionally larger target area, thus encompassing less competition, and as a result increase their arborization areas. Retinal lesions induce ectopic ipsilateral RGC projections Using full eye fills with differently coloured anterograde tracers, we found in anterior and posterior SC regions of α-Del mutant mice individual axon termination patches originating from the ipsilateral eye ( Fig. 2c and Supplementary Fig. S3 ). These patches were localized in the empty territories left by contralateral projections. Early enucleation studies in newborn rats have shown that the removal of the entire input from one eye leads to an extension of ipsilateral projections and influences their laminar targeting in the SC [11] . To examine the topographic and laminar distribution of ipsi- and contralateral RGC projections to the SC in more detail, we analysed coronal and sagittal midbrain sections of α-Del and wild-type control mice after full eye fills with CTB Alexa-488 and -594 ( Fig. 6 ). In wild-type mice, the ipsilaterally projecting RGCs originate in the VTC and map discontinuously in anterior-medial SC [5] , [11] . Their laminar terminations are restricted to the SO, ventral to the terminations of the contralateral projections in the SGS ( Fig. 6b upper panels 1–3). In contrast, sections through the SC of mutant mice revealed that, at P8, ipsilateral projections projecting not only to anterior areas, but also abnormally to posterior locations (Arrows in Fig. 6b , lower panels 1–3). Furthermore, these projections terminate aberrantly in the superficial SGS, at the same level than contralateral projections, leaving the deeper SO empty. The projections from both eyes are completely segregated and do not overlap. This aberrant innervation pattern of ipsilateral axon branches is already visible at earlier stages, during the refinement phase at P4 and remains stable at later stages ( Supplementary Fig. S6 ). 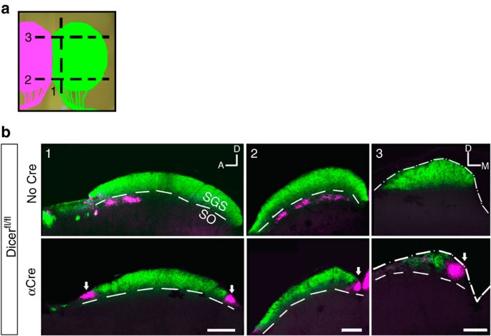Figure 6: Aberrant mapping of ipsilateral RGC axons. (a) Schematic indicating the positions of parasagittal (1) and coronal (2-anterior,3-posterior) sections through the SC depicted in (b) after full eye fills with CTB Alexa-488 (green, contralateral eye) and CTB Alexa-594 (magenta, ipsilateral eye). (b) Sections through the SC of wild-type mice (upper panels) at P8 show the ipsilateral projections (magenta) terminating discontinuously in only anterior positions of the SO below the dorsal-most SGS, which is occupied by contralateral projections (green). In lesion-induced mutant mice, two completely segregated TZs of ipsilateral RGC axons are found in the anterior and posterior SC (arrows). In addition, the terminations are not confined to the deeper SO, but are located incorrectly in the SGS. Dashed lines indicate border between SGS and SO, dashed-dotted lines indicate the dorsal SC border in (3). (n=4 wild-type controls,n=3 α-Del). A, anterior; D, dorsal; M, medial; P, posterior; R, rostral. Scale bar, 200 μm. Figure 6: Aberrant mapping of ipsilateral RGC axons. ( a ) Schematic indicating the positions of parasagittal ( 1 ) and coronal ( 2 -anterior, 3 -posterior) sections through the SC depicted in ( b ) after full eye fills with CTB Alexa-488 (green, contralateral eye) and CTB Alexa-594 (magenta, ipsilateral eye). ( b ) Sections through the SC of wild-type mice (upper panels) at P8 show the ipsilateral projections (magenta) terminating discontinuously in only anterior positions of the SO below the dorsal-most SGS, which is occupied by contralateral projections (green). In lesion-induced mutant mice, two completely segregated TZs of ipsilateral RGC axons are found in the anterior and posterior SC (arrows). In addition, the terminations are not confined to the deeper SO, but are located incorrectly in the SGS. Dashed lines indicate border between SGS and SO, dashed-dotted lines indicate the dorsal SC border in ( 3 ). ( n =4 wild-type controls, n =3 α-Del). A, anterior; D, dorsal; M, medial; P, posterior; R, rostral. Scale bar, 200 μm. Full size image To determine the retinal origin of the aberrant ipsilateral projections in α-Del mutant mice we retrogradely labelled RGCs by unilateral injections of fluorescent microbeads into the SC of P8 animals ( Fig. 7a–d ). Analyses of retinal wholemounts, ipsilateral to injections into anterior SC, show retrogradely labelled RGCs restricted to the ventro-temporal region in both wild-type ( n =3) and mutant mice ( n =3, Fig. 7a ), although more spread out for the latter. As expected, injections into posterior SC did not result in any labelled RGCs in the ipsilateral retina of wild-type mice ( n =6, Fig. 7b ). In contrast, in lesioned mutant mice we found ipsilaterally labelled RGCs not in the VTC, but in nasal retina, which is an appropriate origin for contralateral projections to posterior SC ( n =6, Fig. 7d and Supplementary Fig. S7 ). We hypothesize that these aberrant ipsilaterally projecting RGCs are different from the ones usually generated in the VTC, as all RGCs positive for Zic2, a marker for ipsi-projecting cells in the VTC prenatally [28] , are located inside the Cre-positive retinal area, which is bound to degenerate at perinatal stages ( Fig. 7e–j ). 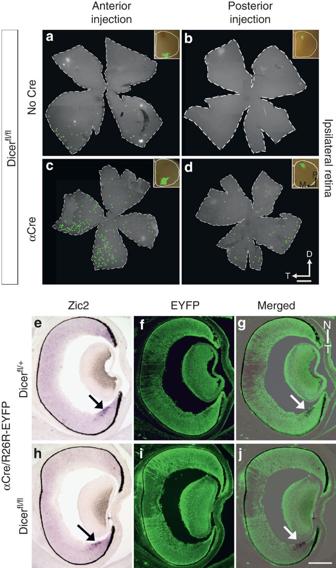Figure 7: The origin of ipsilateral-projecting RGCs is not restricted to the ventral temporal crescent in α-Del animals. (a–d) Whole retina flatmounts detecting RGCs after retrograde labelling using fluorescent microbeads focally injected in the ipsilateral SC of control (a,b) or α-Del mutant mice (c,d) at P8. (a,b) In wild-type controls only injections into anterior ipsilateral SC resulted in retrogradely labelled RGCs in the retina, restricted exclusively to the ventral temporal crescent (VTC) (n=3). No labelled RGCs were detected upon injections in posterior (insets) ipsilateral SC (n=11). (c,d) In α-Del mice injections into both, anterior (c) and posterior (d) ipsilateral SC lead to retrogradely labelled RGCs in the retina. They are generally scattered across the retina, but show a location preference for the ventral temporal retina for anterior injections (c,n=3) and nasal retina for posterior SC injections (d,n=10). (e–j) Panels showin situhybridization using an antisense probe againstZic2(purple) and immunohistochemical detection for EYFP (green) on E16 horizontal retinal sections, from control heterozygous (e,f) and mutant (h,i) mice. Merged images are shown in (g,j). Zic2-positive cells in the VTC (arrow) are located within the Cre-positive (EYFP+) retinal areas, which undergo degeneration in mutant mice at perinatal stages. D, dorsal; N, nasal; T, temporal; VTC, ventral temporal crescent. Scale bar, 500 μm (a,d) and Scale bar, 200 μm (e,j). Figure 7: The origin of ipsilateral-projecting RGCs is not restricted to the ventral temporal crescent in α-Del animals. ( a – d ) Whole retina flatmounts detecting RGCs after retrograde labelling using fluorescent microbeads focally injected in the ipsilateral SC of control ( a , b ) or α-Del mutant mice ( c , d ) at P8. ( a , b ) In wild-type controls only injections into anterior ipsilateral SC resulted in retrogradely labelled RGCs in the retina, restricted exclusively to the ventral temporal crescent (VTC) ( n =3). No labelled RGCs were detected upon injections in posterior (insets) ipsilateral SC ( n =11). ( c , d ) In α-Del mice injections into both, anterior ( c ) and posterior ( d ) ipsilateral SC lead to retrogradely labelled RGCs in the retina. They are generally scattered across the retina, but show a location preference for the ventral temporal retina for anterior injections ( c , n =3) and nasal retina for posterior SC injections ( d , n =10). ( e – j ) Panels show in situ hybridization using an antisense probe against Zic2 (purple) and immunohistochemical detection for EYFP (green) on E16 horizontal retinal sections, from control heterozygous ( e , f ) and mutant ( h , i ) mice. Merged images are shown in ( g , j ). Zic2-positive cells in the VTC (arrow) are located within the Cre-positive (EYFP+) retinal areas, which undergo degeneration in mutant mice at perinatal stages. D, dorsal; N, nasal; T, temporal; VTC, ventral temporal crescent. Scale bar, 500 μm ( a , d ) and Scale bar, 200 μm ( e , j ). Full size image In summary, our results show that upon loss of RGCs in nasal and temporal retina, stable ipsilateral projections are still forming, but both, their origin in the retina and their laminar and topographic distributions in the target are atypical. Here, the ipsilateral map is consistent with arrangements normally appropriate for contralaterally projecting RGCs. The goal of this study was to identify the plasticity potential of the mammalian visual system to respond to perturbations, such as degeneration, during the time when axonal connectivity is established. For this purpose, we generated a genetic mouse model where a defined part of the retina degenerates during the formation of the visual map. Our findings demonstrate the presence of plastic mechanisms in response to such degenerations, with the result to maximise the visual field and its coverage in the brain. In the α-Del mouse line used here, the early expression of Cre-recombinase in progenitor cells in nasal and temporal retina leads to the degeneration of these areas during the first postnatal week [17] , [18] . The Cre-negative central retina, however, remains unaffected. The time window of RGC degeneration at perinatal stages coincides with the formation and maturation of the visual topographic map in mouse [2] . This represents, to our knowledge, for the first time a mouse model with genetically induced and area-specific genetic retinal lesions, to study the consequences of perinatal cells loss on retinotopic connectivity and map formation. In amphibia and fish it has been shown that partial retinal ablations result in a complete recovery of RGC axon afferents in the entire tectum [8] , [10] . This property has been related to the capability of these anamniotes to generate new retinal neurons throughout life due to the presence of retinal stem cells located in the ciliary marginal zone [29] , which are not present in adult mammals [30] . In neonatal rats retinal ablations by mechanical lesions suggested that remaining RGC axons expand partially into deprived SC areas, without clear topographical order [12] . Our findings using a genetically induced retinal lesion show a similar expansion of RGC termination into deprived areas of the SC. There are two important differences, however, first, our data show that the overall retinotopic map is topographically ordered. Second, the extent of the expansion of RGC axon terminations in the SC correlates closely with an expansion of the remaining retinal size. As a result of retinal cells spreading to a larger area, their density is lower. The general ability of RGCs to maintain a retinotopic order in their projections, despite the fact that they originate from an initially narrow stripe in the retina, is consistent with findings that show that mapping is controlled by relative levels of guidance receptors and not absolute values [31] . Therefore, the relative differences of EphA/ephrin-A levels between the nasal and temporal pole of the central stripe is sufficient for appropriate mapping along the caudal-rostral axis of the SC. Our data suggest, however, that this mechanism has its limits. The deprived areas in the very caudal and rostral portions of the SC suggest that the effects mediated by the levels of guidance cues in these areas cannot be overcome. Recent studies have investigated the importance of competitive mechanisms during map formation in mouse using a Math5 mutant model, where only 5% of RGCs are generated [13] . In this model, the few RGC axons originating from across the retina form an incorrect map by targeting the anteromedial SC only, where ephrin-A repulsive guidance cues are the lowest, but medial attractants are the highest. This suggested that axon–axon competition has a role in the correct formation of the topographic map, in addition to molecular cues and activity-dependent mechanisms [13] . This model, however, has some important differences compared with ours. In Math5 mutants, RGC axons experience low axon–axon competition from the time of retinal outgrowth to the SC, leading to an already altered pattern of innervation at birth, before map refinement. In contrast, in our degeneration model all RGC axons are initially innervating the SC and only during the postnatal refinement period the selective loss of RGCs occurs. Therefore, competition is mainly acting on the formation of branches and arborizations and not axon–axon interactions during ingrowth. Although we detect a decrease in density of the remaining wild-type RGCs in the retina, this is much less severe that in the Math5 mutants where 95% of the RGCs are missing [32] . Nevertheless, this lower density of RGCs in our model leads to an expansion of retinal arbours in the SC at topographically appropriate locations. Retinotopic mapping in fish and amphibians does not involve long axon overshoots with subsequent remodelling and is therefore different from map development in higher vertebrates [1] . However, our data suggest that the mammalian system behaves similarly to zebrafish regarding the plasticity of retinal arbours upon changes in innervation density, as it was shown that in zebrafish the innervation of the optic tectum by a single retinal axon increases its branching and arborization area, but without major alterations of the topographic order [14] . Importantly, our retrograde labelling studies show a similar phenotype across the entire SC, not only at the anterior and posterior borders, suggesting a uniform expansion of the map. A normal feature of retinotopic map development is the selective elimination of topographically inappropriate projecting RGCs [33] . The increased distribution of RGCs across the retina that are retrogradely labelled from various positions in the SC could therefore also be, at least in part, a result of reduced eliminations of mistargeted RGCs. Our observation, that the number of remaining (Cre-negative) RGCs is higher in the degenerated retinae as compared with controls, suggests that this is indeed the case. We hypothesize that the reduced elimination of RGCs is based on two possible mechanisms. One is the reduced axon competition discussed above, which allows more RGCs to form stable synapses with collicular targets. The other is directly based on the expansion of the central retinal part after the degeneration of the distal retinal parts. This reshaping of the retina may have a substantial effect on the physical forces that are acting on the individual cells via adherens junctions and compression stress [34] , [35] . Although we cannot measure these forces between retinal cells, our observations that there are significantly less apoptotic cells in Cre-negative retinal areas, and that overall the mutant retinae are thinner than wild-type retinae, are consistent with this hypothesis ( Supplementary Fig. S8 ). These mechanisms leading to the survival of contralaterally projecting RGCs in the remodelled mutant retina, most likely also apply to the uncrossed retinal projection. Normally, RGCs wrongly projecting to the ipsilateral side of the SC are lost during the first postnatal week [11] , [36] . Stable ipsilateral projections originate, in mouse, exclusively in the VTC, an area that lies entirely inside the Cre-positive area in our mutant mouse model. Despite the fact that all VTC RGCs degenerate, we observed stable ipsilateral projections, located in extreme caudal and rostral SC, where contralateral input is absent in our mutants. We assume that the lack of competition enables mistakingly ipsilateral-projecting RGC axons to stabilize their arborizations and protects them from normally occurring removal. In addition, these ipsilateral projections terminate in the SGS, a lamina usually occupied by contralateral visual input only. This incorrect laminar targeting is consistent with earlier findings in rat and hamster, where either the entire input from one eye was removed [11] , [37] or a mechanical retinal lesion was introduced at birth [12] . However, unlike what has been described for experiments using mechanical lesions, the ipsilateral projections in our mutant mice follow a general topographic order, appropriate usually for contralateral projections. This means that, as a consequence, the opposite temporal ends of each eye’s visual field (nasal retinae) map in adjacent positions of the same caudal SC, whereas the central part of the visual field (temporal retina, normally binocular) is represented in the anterior SC ( Fig. 8 ). This therefore represents a change in the opposite map polarity of contra- and ipsilateral projections normally detected in mammals [6] , [38] . 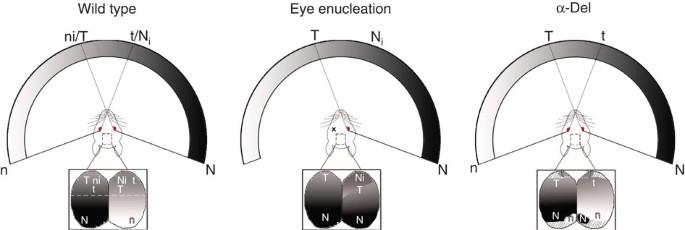Figure 8: Schematic describing the representation of the visual field in the SC in different rodent models. Capitals and lower case letters illustrate zones of the visual field and corresponding retinocollicular projections, which are relative to right and left retina, respectively. The subscript ‘i’ indicates the furthest point of the visual field represented through the nasal border of the ipsilateral-projecting VTC of the retina. In wild-type animals, the zone of binocularity seen by the temporal retina is uniquely represented in the anterior SC so that ipsilateral projections result in an opposing polarity of topographic map (nasal–temporal retina projecting to anterior–posterior SC) relative to contralateral projections (temporal–nasal retina projecting anterior–posterior SC). In animals that undergo eye enucleation at birth, the ipsilateral fibers project continuously in the SC from across the retina with two polarities: an appropriate retinotopic map for normal ipsilateral projections in the anterior SC (nasal–temporal retina projecting anterior–posterior SC) and some aberrant projections in posterior SC by nasal retinal axons. In our genetic lesion mutants (α-Del), contralateral projections form a generally appropriate topographic map, although less refined. In addition, they are unable to innervate the entire SC, leaving an anterior and posterior zone empty. Instead, RGC axons from the ipsilateral eye are occupying some of this empty space and form TZs in anterior and posterior SC, mapping according to contralateral retinotopic polarity. As a result, opposite temporal extremities of the visual fields (‘seen’ by the nasal poles of each retina) map adjacently in the posterior SC. Figure 8: Schematic describing the representation of the visual field in the SC in different rodent models. Capitals and lower case letters illustrate zones of the visual field and corresponding retinocollicular projections, which are relative to right and left retina, respectively. The subscript ‘i’ indicates the furthest point of the visual field represented through the nasal border of the ipsilateral-projecting VTC of the retina. In wild-type animals, the zone of binocularity seen by the temporal retina is uniquely represented in the anterior SC so that ipsilateral projections result in an opposing polarity of topographic map (nasal–temporal retina projecting to anterior–posterior SC) relative to contralateral projections (temporal–nasal retina projecting anterior–posterior SC). In animals that undergo eye enucleation at birth, the ipsilateral fibers project continuously in the SC from across the retina with two polarities: an appropriate retinotopic map for normal ipsilateral projections in the anterior SC (nasal–temporal retina projecting anterior–posterior SC) and some aberrant projections in posterior SC by nasal retinal axons. In our genetic lesion mutants (α-Del), contralateral projections form a generally appropriate topographic map, although less refined. In addition, they are unable to innervate the entire SC, leaving an anterior and posterior zone empty. Instead, RGC axons from the ipsilateral eye are occupying some of this empty space and form TZs in anterior and posterior SC, mapping according to contralateral retinotopic polarity. As a result, opposite temporal extremities of the visual fields (‘seen’ by the nasal poles of each retina) map adjacently in the posterior SC. Full size image In summary, our findings show that the retina is able to respond to tissue and cell loss at perinatal stages, increasing its remaining area and the number of surviving RGCs. Previous computational models on retinotopic map development only partially fit our data [39] , [40] , [41] , [42] . However, none of these approaches considered plastic changes of the retina itself, such as we reported here. It will be therefore interesting to use our data as a basis to adapt and re-validate in-silico modelling of visual map dynamics. We provide evidence for a plastic response to counterbalance the effects of the nasal and temporal retinal degeneration resulting in partial recovery of the visual field and the maintenance of a homogeneous retinotopic map. These effects may be reached through several mechanisms in parallel, such as retina expansion, changes in cell survival and expansion of RGC axonal arbours, but with the cost of reduced retinal cell density and topographic precision. How other parts of the nervous system respond to the changed innervation patterns in the SC, for example, projections from the visual cortex to the aberrantly located ipsilateral terminations, is an important question for the future. Animals All animal procedures were carried out according to institutional guidelines and protocols approved by the KCL Ethics Committee and the UK Home Office. Floxed Dicer1 mice [15] were purchased from The Jackson Laboratory. Pax6αCre mice [16] were kindly provided from D. O’Leary (Salk Institute, USA). R26R-EYFP mice [23] were kindly provided by Albert Basson (King’s College). Mice with degenerated nasal and temporal areas of the retina (αCre;Dicer fl/fl ) are referred to as α-Del mutant mice in the text. As controls, we used either mice heterozygous for Dicer (Dicer fl/+ and Cre-positive ) or Cre-negative mice (Dicer fl/fl or Dicer fl/+ ). Genotyping was performed by PCR according to The Jackson Laboratory guidelines (Dicer fl/fl and R26R-EYFP mice) and Marquardt et al . [16] (αCre mice). Anterograde and retrograde labelling Mice were anesthetized with a mix of oxygen-isoflurane. Pulled glass micropipettes and Picospritzer III were used for the injections. Anterograde labelling was performed by full eye fills of CTB conjugated to Alexa- 488 or Alexa 594 (Invitrogen). The following day, mice were perfused with 4% PFA under terminal anaesthesia. Brains were recovered and postfixed in 4% PFA solution at 4 °C until sectioning on a vibratome. Retrograde labelling was performed by injection of green and red microbeads (Retrobeads, Lumafluor) in the SC of P7 mice. Up to 24 h later, mice were perfused with 4% PFA; after postfixing, retinae were removed and flatmounted for imaging. Focal injections into the retina were performed using 1,1′-dioctadecyl-3,3,3′,3′-tetramethylindocarbocyanine perchlorate (DiI) as previously described [2] . Immunohistochemistry Fixed tissue was cryosectioned and used for immunohistochemistry as previously described [43] . Primary antibodies against GFP (1:500, Abcam 13970), Brn3a (1:500, Millipore MAB 1585), Caspase-3 (1:500, Abcam 13847), Ki67 (1:500, Abcam 15580) were visualized with species-specific secondary antibodies, conjugated to Alexa-488 and Alexa-594 (Invitrogen). Sections were counterstained Hoechst (1:2,000, molecular probes). Whole-mount staining of retinae, chiasm and SC was as for sections but with extended washing and incubation times. In situ hybridization DIG-labelled riboprobes were prepared using the DIG-RNA labelling kit (Roche) and cDNAs encoding Foxg1 (0.9 kb), Foxd1 (1.3 Kb), EphA5 (0.5 kb), EphA6 (0.6 kb), EphrinA5 (0.3 kb) and Zic2 (0.7 kb) subcloned in pBluescript SK vector. In situ hybridization was performed on defrosted cryosections treated with HCl 0.2 N (in DEPC water) for tissue permeabilization and acetic anhydride (0.2% vol/vol) in triethanolamine 0.1 M (in DEPC water) in order to decrease background. Prehybridization was carried out for 90 min at 65 °C in hybridization mix (50% vol/vol Formamide, SSC 5X, yeast tRNA 10 mg ml −1 , Heparin 10 mg ml −1 , 0.5% v/v Tween in DEPC water). Five microlitre of probe mix (0.3 μg μl −1 , obtained upon transcription) for 1 ml of hybridization mix was used during the hybridization step carried out overnight at 65 °C. Next day stringency washing were performed at 65 °C in formamide (50% v/v) and SSC (5X) for 2 h. Probe detection was carried out using AP-conjugated anti-DIG antibody incubated overnight (1:2000, Roche) followed by colour reaction using NBT-BCIP (Roche). Tissue sectioning and Imaging Fixed tissues were equilibrated in 30% sucrose w/vol and stored at −80 °C. Cryosectioning was carried out at 20 μm (immunostaining) and 14 μm ( in situ hybridization). Vibratome sectioning of CTB-Alexa injected brains was performed on fixed tissue at 100 μm. Imaging of CTB-Alexa labelled whole-mount SC was performed with a Leica Stereomicroscope M165FC connected to a Qimaging CCD colour camera and Volocity Acquisition software (Perkin-Elmer). Because of the thickness of the tissue (>4 mm), the relatively large depth of field and our intension to avoid signal loss from sparse axonal terminations, images appear overexposed for most of the SC. However, detailed analyses (with lower exposure times) on these samples were performed upon vibratome sectioning of the SC using confocal imaging. Imaging of retina cryosections after in situ hybridization/immunohistochemistry and whole flatmounted retrogradelly labelled retinae was performed with a Zeiss Axioskop connected to a cooled monochrome CCD camera (Retiga EXi Blue) and Volocity acquisition software. Superior colliculi of focally injected mice and vibratome sections of anterogradely labelled SC with CTB-Alexa were imaged with a confocal microscope Nikon Eclipse 80i using 360 μm Z-stacks starting from the SC surface (20 stacks, 18 μm). Image and data processing Quantification of caspase-3 and Ki-67-positive cells was performed on five fields for each genotype (four animals for each genotype/stage). For Supplementary Fig. S2 , only cells positive for Casp-3 and YFP were considered for calculation. For Fig. 4 , only cells in the ganglion cell layer and neuroblastic layer of Cre-negative area were considered for calculation Casp-3 and Ki-67, respectively. Quantification of Brn3a-positive cells was performed on five retinae for each genotype at P8 and four retinae for each genotype at P0. One field at × 40 magnification as shown by insets for each pole of the retina plus a field from centre retina (five fields for each retina in total) were sampled for calculation. At P8, RGCs density was calculated as density average of Brn3a-positive cells observed in the five different high magnification fields (shown in figure insets) and rounding off the density differences present among the central and the peripheral retina. At P0, RGCs density was calculated as density average of Brn3a-positive cells observed either in the fields from αCre-positive or -negative zones (four fields for each zone per retina). The total numbers of RGCs were calculated multiplying the RGC densities with the retinal areas (P8) or αCre + +/− zones (P0). Retinal areas were measured using ImageJ. Quantification of αCre + positive surfaces in Dicer fl/fl and control retinae and SC was performed using ImageJ. Borders of the SC were manually traced according to bright fields images. All retinae and SCs were imaged through fields acquired with a low magnification (× 5) objective on Zeiss Axioskop microscope connected to monochrome CCD camera (Retiga EXi Blue) and mounted using Photoshop CS3. Images were adjusted for contrast and brightness using Photoshop CS3. Retrogradely labelled RGCs were marked on retinal images with camera lucida using high magnification. Quantification of dispersion of retrogradely labelled RGCs was performed using Photoshop CS3 dividing the retinae in 6 concentric circles. ImageJ was used to count cells and calculating surfaces. Injections made in anterior, central and posterior SC were pooled for calculation ( n =13 for both genotypes). All analysis was done blind to genotype. Data were analysed using Sigmaplot 12 and Excel and reported as in the main text. How to cite this article: Maiorano, N. A. et al . Restricted perinatal retinal degeneration induces retina reshaping and correlated structural rearrangement of the retinotopic map. Nat. Commun. 4:1938 doi: 10.1038/ncomms2926 (2013).